DNA unmethylome profiling by covalent capture of CpG sites Dynamic patterns of cytosine-5 methylation and successive hydroxylation are part of epigenetic regulation in eukaryotes, including humans, which contributes to normal phenotypic variation and disease risk. Here we present an approach for the mapping of unmodified regions of the genome, which we call the unmethylome. Our technique is based on DNA methyltransferase-directed transfer of activated groups and covalent biotin tagging of unmodified CpG sites followed by affinity enrichment and interrogation on tiling microarrays or next generation sequencing. Control experiments and pilot studies of human genomic DNA from cultured cells and tissues demonstrate that, along with providing a unique cross-section through the chemical landscape of the epigenome, the methyltransferase-directed transfer of activated groups-based approach offers high precision and robustness as compared with existing affinity-based techniques. DNA cytosine-5 methylation is a widespread epigenetic mark in high eukaryotes including mammals. DNA methylation profiles are highly variable across different genetic loci, cells and organisms, and are dependent on tissue, age, sex, diet and disease [1] , [2] . In somatic cells, 5-methylcytosine (5mC) is largely restricted to CpG sites [3] . Recent studies of vertebrate DNA found that 5mC residues can undergo oxidation to 5-hydroxymethylcytosine (hmC), 5-formylcytosine (fC) or 5-carboxycytosine (caC) in a tissue- and locus-specific manner [4] . Existing approaches for the determination of the modification status of CpG sites are largely based on detection of 5mC and can be divided into bisulfite conversion-based methods, affinity capture-based techniques and restriction endonuclease-based methods [5] , [6] , [7] , [8] . The gold standard is bisulfite conversion coupled with sequencing due to its ability to map 5-modified cytosines at a single-base resolution [9] , [10] . However, bisulfite conversion displays fC and caC as unmodified C, and discrimination between 5mC and hmC requires additional cumbersome pretreatment steps [11] , [12] . Overall, it is a labour-intensive technique [3] , [13] that is still prohibitively expensive for large-scale populational studies. In affinity enrichment methods, methylated DNA fragments are non-covalently bound to 5mC-antibodies (MeDIP) [6] or to the methyl-CpG binding domain of MBD2 or MeCP2 (refs 14 , 15 ). The latter methods suffer from a poor coverage of the medium to low CpG density regions of the genome [16] , [17] . Restriction enzyme-based approaches permit interrogation of either the unmodified or modified fraction of genomic DNA (gDNA) [5] , [8] , [18] , [19] , [20] , [21] , however, their coverage and resolution is inherently limited by the sequence- and modification-type-specificity of available enzymes. Therefore, none of the existing methods alone is able to grasp the breath and chemical complexity of the mammalian epigenome. To circumvent these limitations, we pursued a novel strategy for determining the genome modification status that is based on covalent labelling of unmodified CpG sites. Targeted labelling of DNA was achieved by using a recently devised chemo-enzymatic approach named ‘methyltransferase-directed transfer of activated groups’ (mTAG) [22] followed by chemoselective biotinylation of the attached terminal amine or azide groups. The labelled genomic fragments were selectively enriched on streptavidin beads and analysed on tiling microarrays and next generation sequencing. Studies of human gDNA from cultured cells and tissues demonstrate that this technique offers nanogram sensitivity, as well as high precision and reproducibility. Notably, we demonstrate that mTAG-based methods uniquely permit a positive identification of unmethylated loci in various complex genomic contexts such as repeat sequences and partially methylated regions. General approach for covalent capture of genomic CpG sites Previously, we demonstrated that the HhaI DNA cytosine-5 methyltransferase, which serves as a structural and mechanistic paradigm for this class of enzymes, can be engineered to direct efficient transfer of extended linear groups from synthetic AdoMet analogues onto the GCGC sites in DNA [23] , [24] . Following this concept, we engineered the CpG-specific cytosine-5 MTase SssI (M.SssI) [25] , by site directed mutagenesis of two conserved positions in the cofactor-binding pocket (Q142A/N370A). The recombinant His-tagged protein was expressed in E. coli and isolated in an AdoMet-free form ( Supplementary Methods ). We have also synthesized a series of optimized AdoMet analogues that contain a sulfonium-bound 6-substituted hex-2-ynyl side chain [26] . The engineered M.SssI (eM.SssI) exhibited a higher than 100-fold increase in the alkylation activity with these synthetic cofactors ( Supplementary Fig. S1 ) as compared with native M.SssI. As the MTase-directed reactions are highly specific with respect to the target sequence, modified residue and atomic position [22] , [27] , the M.SssI-directed mTAG labelling selectively tags all unmodified and hemimethylated CpG sites [25] and excludes methylated target sites (5mCpG) in gDNA. In this study, two biotin conjugation chemistries were explored ( Fig. 1b ). In the first series, conventional chemoselective coupling of a primary alifatic amine group, which are absent from native DNA, with a biotin probe carrying an N -hydroxysuccinimide (NHS) group was employed ( Supplementary Fig. S2 ). Alternatively, we used a fully bioorthogonal copper-free click-chemistry, namely Huisgen 1,3-dipolar cycloaddition of azide to a ring-activated alkyne, dibenzocyclooctyne group (DBCO) [28] . In both cases, a biotin linker containing a cleavable S-S bond was present to facilitate the detachment of the captured DNA fragments. 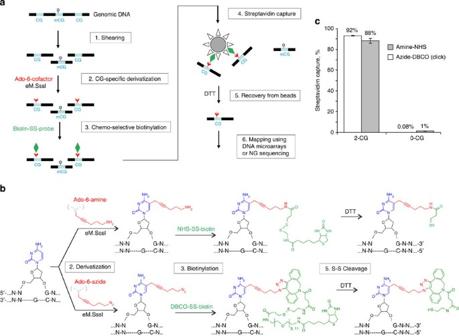Figure 1: mTAG labelling-based enrichment and analysis of unmethylated CpG sites in the genome. (a) Flow diagram of the analytical procedure. gDNA is randomly sheared to short fragments (Step 1) and treated with an engineered SssI DNA methyltransferase (eM.SssI) and a cofactor analogue (Ado-6-amine or azide) to attach reactive groups to unmodified CpG sites (Step 2). The derivatized target sites are biotin-tagged usingN-hydroxysuccinimidyl ester (Biotin-SS-NHS) (Step 3) and labelled fragments are selectively captured on streptavidin-coated magnetic beads (Step 4). Bound DNA fragments are recovered by cleavage of a disulphide bond in the biotin linker with DTT (Step 5). The enriched fragments are ligated to adaptors and PCR-amplified (Step 6) for microarray analysis or DNA sequencing (Step 7). (b) Covalent transformations during derivatization, biotin tagging and linker cleavage (Steps 2, 3 and 5) using amine-NHS (upper) or azide-DBCO (lower) conjugation chemistries (one of the two triazol regioisomers formed in Step 3 is shown); (c) Affinity capture of DNA fragments containing unmodified CpG sites. Reference DNA fragments, containing two or no CpG sites (2-CG and 0-CG, respectively) was each combined with 300 ng of sonicated human gDNA and processed as described (Steps 1–4) using the amine or azide conjugation chemistries as indicated. The efficiency of CpG capture is assessed by on-beads qPCR analysis of the reference DNA fragments. Error bars defined as ±s.d. from duplicate experiments. Figure 1: mTAG labelling-based enrichment and analysis of unmethylated CpG sites in the genome. ( a ) Flow diagram of the analytical procedure. gDNA is randomly sheared to short fragments (Step 1) and treated with an engineered SssI DNA methyltransferase (eM.SssI) and a cofactor analogue (Ado-6-amine or azide) to attach reactive groups to unmodified CpG sites (Step 2). The derivatized target sites are biotin-tagged using N -hydroxysuccinimidyl ester (Biotin-SS-NHS) (Step 3) and labelled fragments are selectively captured on streptavidin-coated magnetic beads (Step 4). Bound DNA fragments are recovered by cleavage of a disulphide bond in the biotin linker with DTT (Step 5). The enriched fragments are ligated to adaptors and PCR-amplified (Step 6) for microarray analysis or DNA sequencing (Step 7). ( b ) Covalent transformations during derivatization, biotin tagging and linker cleavage (Steps 2, 3 and 5) using amine-NHS (upper) or azide-DBCO (lower) conjugation chemistries (one of the two triazol regioisomers formed in Step 3 is shown); ( c ) Affinity capture of DNA fragments containing unmodified CpG sites. Reference DNA fragments, containing two or no CpG sites (2-CG and 0-CG, respectively) was each combined with 300 ng of sonicated human gDNA and processed as described (Steps 1–4) using the amine or azide conjugation chemistries as indicated. The efficiency of CpG capture is assessed by on-beads qPCR analysis of the reference DNA fragments. Error bars defined as ±s.d. from duplicate experiments. Full size image mTAG labelling using amine-NHS chemistry The general procedure for the enrichment of unmodified DNA consisted of five steps ( Fig. 1a ). Human gDNA was sonicated to yield short (50–300 bp) fragments (Step 1), aminoalkylated with eM.SssI and Ado-6-amine (Step 2), biotinylated with an amino-reactive reagent NHS-SS-biotin (Step 3) and captured on streptavidin beads (Step 4). In our initial control experiments that measured the levels of labelling and DNA capture (Steps 2–4) by quantitative PCR (qPCR), we designed a series of 200–230 bp DNA fragments containing none, 1, 2 or 4 unmodified CpG sites (probes 0-CG, 1-CG, 2-CG and 4-CG, respectively; Fig. 2a ). These DNA fragments were tested individually and as spike-ins to sonicated gDNA samples. Robust mTAG labelling produced CpG capture efficiencies around 90%, whereas a 0-CG spike was detectable at a level of ~1% ( Fig. 1c ). In subsequent experiments designed to optimize the procedure, three levels of mTAG labelling intensity (as determined by the streptavidin capture efficiency of the 2-CG probe) were explored: 5–10% capture-low labelling; 20–35% capture-medium labelling; 60–80% capture-high labelling. It was found that, at medium labelling, the capture of the model DNA fragments linearly correlated with the number of unmodified CpG sites ( Fig. 2b ), an effect that persisted in the presence of methylated DNA fragments ( Supplementary Fig. S3 ) and upon deep dilution with native gDNA ( Fig. 2c ). Efficient recovery of streptavidin-bound DNA (Step 5) was achieved via mild chemical cleavage of a disulphide bond in the biotin connector with dithiothreitol (DTT). The released DNA fragments retain only a part of the original linear side chain attached to the labelled cytosine residues ( Fig. 1b and Supplementary Fig. S2 ), which did not interfere with downstream PCR amplification ( Supplementary Fig. S4 ). 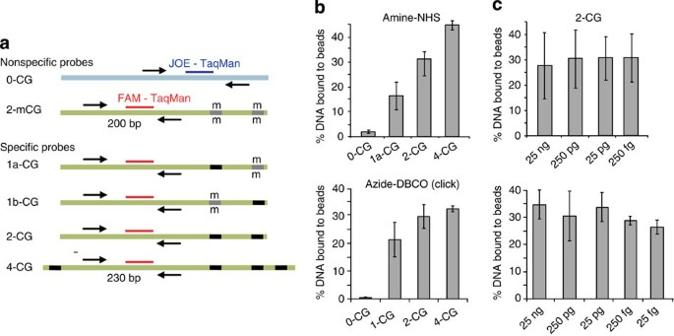Figure 2: Streptavidin capture of unmodified CpG sites in model DNA fragments. (a) Schematic of nonspecific (containing no CpG sites, 0-CG) and specific (containing 1, 2 or 4 CpG sites) DNA probes derived from the mouse genome for quantification of DNA using TaqMan qPCR. CpG sites are shown in black and locations of qPCR primers are shown as arrows. ‘m‘ denotes a premethylated CpG site. (b) DNA recovery through Steps 1–4. DNA probes (25 ng) as indicated were combined with 300 ng of sheared and blunt-ended gDNA and then mTAG-labelled at Medium Intensity (top, amine-NHS conjugation chemistry; bottom, azide-DBCO conjugation chemistry). DNA was further processed as described in Methods and the amount of captured DNA was determined in qPCR analysis. (c) DNA recovery through Steps 1–4 in a series of 10-fold dilutions (1:10–1:1,000,000). A specified amount of the 2-CG probe was combined with 300 ng of sheared gDNA and mTAG-labelled at Medium Intensity (top, amine-NHS conjugation chemistry; bottom, azide-DBCO conjugation chemistry). DNA was further processed as described and the amount of captured DNA was determined by qPCR analysis. Error bars defined as ±s.d. from duplicate experiments. Figure 2: Streptavidin capture of unmodified CpG sites in model DNA fragments. ( a ) Schematic of nonspecific (containing no CpG sites, 0-CG) and specific (containing 1, 2 or 4 CpG sites) DNA probes derived from the mouse genome for quantification of DNA using TaqMan qPCR. CpG sites are shown in black and locations of qPCR primers are shown as arrows. ‘m‘ denotes a premethylated CpG site. ( b ) DNA recovery through Steps 1–4. DNA probes (25 ng) as indicated were combined with 300 ng of sheared and blunt-ended gDNA and then mTAG-labelled at Medium Intensity (top, amine-NHS conjugation chemistry; bottom, azide-DBCO conjugation chemistry). DNA was further processed as described in Methods and the amount of captured DNA was determined in qPCR analysis. ( c ) DNA recovery through Steps 1–4 in a series of 10-fold dilutions (1:10–1:1,000,000). A specified amount of the 2-CG probe was combined with 300 ng of sheared gDNA and mTAG-labelled at Medium Intensity (top, amine-NHS conjugation chemistry; bottom, azide-DBCO conjugation chemistry). DNA was further processed as described and the amount of captured DNA was determined by qPCR analysis. Error bars defined as ±s.d. from duplicate experiments. Full size image To assess the performance of this new technology for epigenome studies, we carried out further control experiments with sheared human gDNA in which all cytosine modifications were stripped by PCR amplification. These ‘fully unmodified’ DNA samples were mTAG-labelled, with separate aliquots for the low, medium and high labelling intensities and bound to streptavidin beads. The enriched DNA samples were PCR-amplified and analysed on a human genome tiling microarray (E array covering chromosomes 5, 7 and 16 from the Affymetrix 2.0 R whole-genome human tilling microarray set). Probe intensities for chromosome 5 (2.6 million probes covering 1,013 genes and 1,227 CpG islands) were scale normalized and averaged. Optimal performance was again observed at the medium labelling intensity of around 25%, although in general, variations in the range of 10–80% showed rather small changes in the mean signal profile ( Fig. 3a ). The relationship of the mean log array signal intensity versus the local CpG density was linear ( r =0.99) in the range from 0 to 10 unmethylated CpG sites per 200 bp fragment ( Fig. 3a ), and then reached a plateau at higher CpG densities. Given that 87% of the genome contains 10 or less CpGs per 200 bp ( Fig. 3b ) and only 20–30% of CpGs are unmodified [29] , the overwhelming majority of native gDNA fragments should fall within the linear mTAG labelling and interrogation range. 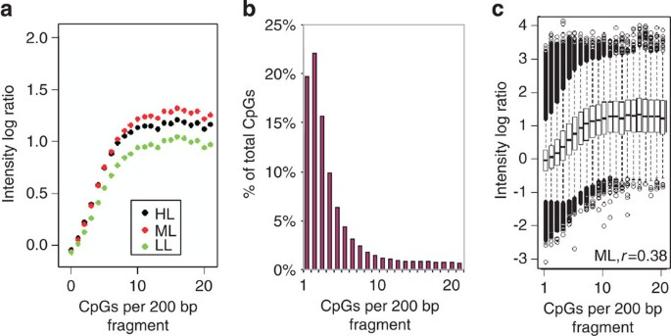Figure 3: Microarray analysis of mTAG-based enrichment of modification-devoid gDNA. Modification-devoid human gDNA (prepared by ligating double-stranded adaptors to sheared gDNA, followed by PCR amplification for 15 cycles as described in Methods) was mTAG-labelled using amine-NHS chemistry at different labelling intensities (low labelling intensity, LL; medium labelling intensity, ML; high labelling intensity, HL), enriched on streptavidin beads and analysed on DNA microarrays representing chr 5. (a) Mean log ratios of microarray intensities, normalized to unlabelled control (0% labelling intensity) and plotted against the number of CpG sites in 200 bp-sized windows. (b) Distribution of CpG sites in 200 bp fragments of different CpG content on human chromosome 5. (c) Box diagram of the array intensity log ratios for a ML experiment plotted against the number of CpG target sites. The bottom and the top of boxes define the first and third quartiles, whiskers mark the lowest and highest data points that are within a 1.5-fold interquartile range. Figure 3: Microarray analysis of mTAG-based enrichment of modification-devoid gDNA. Modification-devoid human gDNA (prepared by ligating double-stranded adaptors to sheared gDNA, followed by PCR amplification for 15 cycles as described in Methods) was mTAG-labelled using amine-NHS chemistry at different labelling intensities (low labelling intensity, LL; medium labelling intensity, ML; high labelling intensity, HL), enriched on streptavidin beads and analysed on DNA microarrays representing chr 5. ( a ) Mean log ratios of microarray intensities, normalized to unlabelled control (0% labelling intensity) and plotted against the number of CpG sites in 200 bp-sized windows. ( b ) Distribution of CpG sites in 200 bp fragments of different CpG content on human chromosome 5. ( c ) Box diagram of the array intensity log ratios for a ML experiment plotted against the number of CpG target sites. The bottom and the top of boxes define the first and third quartiles, whiskers mark the lowest and highest data points that are within a 1.5-fold interquartile range. Full size image Next, we analysed native gDNA samples using mTAG-based enrichment coupled with interrogation on tiling arrays (mTAG-chip). mTAG enrichment of the DNA unmethylome from human tissues showed low technical variation (typical correlations in the range of 0.89–0.93). Analysis of the mTAG-chip profiles consistently detected known unmethylated genomic regions ( Supplementary Fig. S5 ) that showed strong associations with histone acetylation and H3K4 methylation—marks of active promoters and functional enhancers [30] ( Supplementary Fig. S6 ). We also performed a rigorous quantitative comparison of the mTAG approach with published data sets from methylation-sensitive restriction enzyme sequencing (MRE-seq), MBD-seq and MeDIP-seq experiments [8] using IMR90 and H1 MethylC-seq maps [3] as the gold standard. For this, fetal lung fibroblast (IMR90) gDNA (gift of R. Lister) was assessed in the mTAG procedure. Correlation analyses with the IMR90 MethylC-seq map at sequencing depths of >5, >10 or >15 reads (with effective genome coverage of 62%, 35% and 19%, respectively) were carried out for 1,000, 400 or 200 bp-sized windows and were stratified across deciles of local CpG densities ( Fig. 4a ; Supplementary Fig. S7 ). Depending on the decile, correlation coefficients varied from 0.14 to 0.31 ( Fig. 4a ). In MRE-seq, MBD-seq and MeDIP-seq experiments on H1 human embryonic stem cells [3] with the corresponding reference MethylC-seq map [8] , we found correlations to be close to 0, except at the highest CpG density decile ( Fig. 4a ). Altogether, mTAG-chip proved superior to the other methods in 8 or even 9 CpG density deciles representing 80–90% of the human genome and 50–68% of all CpGs ( Supplementary Table S2 ). Similarly, a concordance analysis showed that mTAG-chip achieves better parameters than MeDIP-chip ( Fig. 4b ). Notably, the overall precision in mapping the DNA methylome increases significantly in an ‘integrative’ mTAG/MeDIP-chip experiment, even in the regions of higher CpG density, where both techniques are similarly faithful. 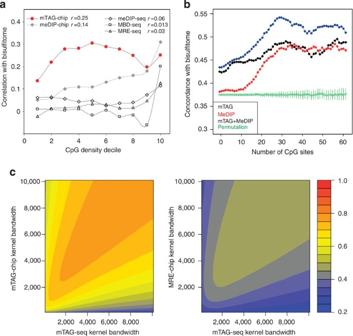Figure 4: Comparison of the mTAG approach with existing methylome profiling methods. (a) Pearson correlations between experimental mTAG-chip (amine-NHS chemistry), MeDIP-chip of IMR90 gDNA and published data of MeDIP-seq, MBD-seq, MRE-seq analysis of H1 gDNA8were determined for 1 kb tiles on chr4 against the corresponding MethylC-seq data3and stratified according to local CpG density. Mean log ratios of probes for chip data or mean numbers of reads for seq data in the tiles were calculated and correlated to mean methylation scores of the MethylC-seq data (minimum 10 reads) using Pearson correlation. Missing-value tiles were excluded, and non-CG methylation sites in the H1 MethylC-seq data were removed before averaging and correlation with the MRE-seq and MBD-seq data. Aggregate correlation numbers (r) obtained with each analytical procedure are shown above the plots. (b) Three-way concordance analysis of mTAG-chip and MeDIP-chip approaches with MethylC-seq. Mean log ratios of the probes in 1 kb tiles were calculated and a methylation type of a tile defined as follows: weak methylation ?25% of the signal distribution; partial methylation=25%<signal<75% of the signal distribution; high methylation=signal>75% of the signal distribution. Concordance with the bisulfitome data (at >5 reads) covering human chr4+chr15+chr18 was determined if the type matched with that of the MethylC-seq call; random calls give a concordance of ~0.375. Data stratified according to the number of CpG sites per tile. (c) Correlation of mTAG-chip and MRE-chip versus mTAG-seq using Gaussian kernel smoothing. Gaussian kernel smoothing was used to examine Pearson correlations between mTAG-seq and mTAG-chip (click chemistry) or MRE-chip data representing human brain DNA unmethylomes. In both cases, the correlation increases with increased kernel bandwidth until it reaches a plateau at a bandwidth of around 1.9 kb for mTAG-seq and 3.1 kb for mTAG-chip data. Figure 4: Comparison of the mTAG approach with existing methylome profiling methods. ( a ) Pearson correlations between experimental mTAG-chip (amine-NHS chemistry), MeDIP-chip of IMR90 gDNA and published data of MeDIP-seq, MBD-seq, MRE-seq analysis of H1 gDNA [8] were determined for 1 kb tiles on chr4 against the corresponding MethylC-seq data [3] and stratified according to local CpG density. Mean log ratios of probes for chip data or mean numbers of reads for seq data in the tiles were calculated and correlated to mean methylation scores of the MethylC-seq data (minimum 10 reads) using Pearson correlation. Missing-value tiles were excluded, and non-CG methylation sites in the H1 MethylC-seq data were removed before averaging and correlation with the MRE-seq and MBD-seq data. Aggregate correlation numbers ( r ) obtained with each analytical procedure are shown above the plots. ( b ) Three-way concordance analysis of mTAG-chip and MeDIP-chip approaches with MethylC-seq. Mean log ratios of the probes in 1 kb tiles were calculated and a methylation type of a tile defined as follows: weak methylation ?25% of the signal distribution; partial methylation=25%<signal<75% of the signal distribution; high methylation=signal>75% of the signal distribution. Concordance with the bisulfitome data (at >5 reads) covering human chr4+chr15+chr18 was determined if the type matched with that of the MethylC-seq call; random calls give a concordance of ~0.375. Data stratified according to the number of CpG sites per tile. ( c ) Correlation of mTAG-chip and MRE-chip versus mTAG-seq using Gaussian kernel smoothing. Gaussian kernel smoothing was used to examine Pearson correlations between mTAG-seq and mTAG-chip (click chemistry) or MRE-chip data representing human brain DNA unmethylomes. In both cases, the correlation increases with increased kernel bandwidth until it reaches a plateau at a bandwidth of around 1.9 kb for mTAG-seq and 3.1 kb for mTAG-chip data. Full size image The large difference in correlation between mTAG-chip and the MRE-, MeDIP- and MBD-sequencing-based methods prompted us to verify if the observed differences arose because of distinct platforms. We therefore performed DNA methylome analysis of the IMR90 gDNA using MeDIP-chip. The observed MeDIP-chip correlations were lower than the ones of the mTAG-chip, however, the former showed significantly higher correlations to MethylC-seq in comparison to the MRE-seq, MBD-seq and MeDIP-seq data sets ( Fig. 4a ; Supplementary Fig. S7 ). The reasons for the low correlation (<0.4) between the MethylC-seq and the enriched microarray and sequencing-based data sets were not completely clear. In part, it may derive from an insufficient x-fold coverage of the methylome in the MethylC-seq experiment (only 19% of the genome covered at >15 reads), which is required to offset an inherent unevenness of DNA sequencing [31] . Depending on the degree of intra-individual variation of DNA modification, the minimal coverage may vary dramatically from locus to locus and may often require as many as 50–60 reads [32] . mTAG labelling using azide-alkyne cycloaddition In the second part of the study, we introduced a bioorthogonal copper-free click-reaction [28] for mTAG labelling ( Fig. 1b , bottom). The analytical procedure remained essentially the same, except that a different AdoMet analogue (Ado-6-azide, Supplementary Fig. S1a ) and a matching biotin reagent (DBCO-SS-biotin) were used in Step 2 and Step 3 ( Fig. 1a ), respectively. Control qPCR experiments using the 200–230 bp DNA fragments showed a nearly identical labelling efficiency but offered a 10-fold reduced background labelling as compared with the previous conjugation ( Fig. 1c ). Other technical parameters appeared identical with both chemistries ( Fig. 2 ; Supplementary Fig. S3 ) except that amplification of the enriched fragments after chemical cleavage from the beads was slightly reduced in the latter approach (20–25% drop in amplification efficacy over two targets sites modified at High labelling intensity, Supplementary Fig. S4 ). At Medium labelling intensity, an effect of similar magnitude would be expected for fragments containing many (>4) unmethylated CpG sites. This slight impairment most likely derives from the fact that a larger chemical group remains attached to the DNA after the chemical cleavage of the S-S bond in the biotin linker ( Fig. 1b ), which may impede a DNA polymerase during the initial cycles of PCR. However, no detectable gross effect was reported in the case of TAB-seq [12] and TAmC-seq [33] methods in which an even bulkier linker group (glucose-azide-DBCO) remained in the released DNA. We further adapted the Click version of mTAG for large-scale studies using a 96-well plate format ( Supplementary Methods ). We then analysed mTAG-enriched gDNA samples on the microarrays. Comparisons between mTAG-chip and MeDIP-chip were made using gDNA from human brain and sperm. In our hands, samples enriched with the mTAG technique displayed better hierarchical clustering than MeDIP-enriched samples ( Supplementary Fig. S8 ). The MeDIP and mTAG technique target different CG sites, methylated and unmodified, respectively. This was confirmed in a tiling microarray experiment examining chromosomes 10, 13, 14 and 17. As expected, negative correlations were observed in the brain ( r =−0.52) and sperm ( r =−0.35) samples between mTAG and MeDIP-chip probes with high signal intensities. It was previously shown that certain bacterial C5-MTases can catalyse sequence-specific removal of the 5-hydroxymethyl group from a hmC residue yielding unmodified C [34] . If this also occurs under conditions of mTAG labelling of gDNA, the dehydroxymethylated CpG will be spuriously labelled as unmodified cytosine, and enriched. In control experiments with a PCR-generated 190 bp DNA fragment containing a single modified CpG site, a low amount of labelling was detected at the hmC, which became negligible in a reaction with pH=6.5 ( Supplementary Fig. S9 ). To examine if this side reaction creates a measurable difference in human brain gDNA, which exhibits higher hmC content compared with other tissues [35] , [36] , the DNA was treated with M.SssI for an extended period of time. hmC sites were measured before and after M.SssI treatment using an assay where hmC glucosylation was coupled with MspI restriction enzyme digestion [37] . The microarray data (chromosome 1 and 6, Supplementary Fig. S10 ) showed that the number of hmC sites detected in M.SssI-exposed and control samples is the same within error, suggesting a negligible, if any, contribution of this side reaction to genomic analyses. Although caC sites also show some labelling in control experiments ( Supplementary Fig. S9 ), their extremely low abundance in gDNA [36] should not affect routine epigenomic studies. We further assessed DNA unmethylome profiles in the post-mortem human brain using the mTAG-seq approach. In this experiment ~100 million reads per sample were generated. Biological and technical replicates showed similarity but were clearly distinct from a non-enriched control in all validation measures, including epigenome-wide pairwise correlation, mapping statistics, standard browser and whole-chromosome profiles ( Supplementary Figs S11–S14 ). The mTAG-seq results were also globally compared with those of mTAG-chip and MRE-chip experiments performed on the same brain gDNA samples. We used Gaussian kernel smoothing, which takes into account regional DNA modification effects, and detected that correlation between the microarray and mTAG-seq data sets gradually increased and reached a maximum ( r = 0.78 and 0.49 for mTAG-chip and MRE-chip, respectively) when the size of the kernel bandwidth expanded to 1.9 kb for mTAG-seq and 3.1 kb for the mTAG-chip data ( Fig. 4c ). The kernel bandwidths in the mTAG-seq and mTAG-chip experiment distributed 50% of its weight in a window of ~1 and ~1.5 kb, respectively, which likely reflects an inherent 1–2 kb CpG co-methylation in the human genome [38] . mTAG-seq and mTAG-chip correlation coefficients varied for different GC content regions ( r =0.47, 0.85 and 0.75 for probes with low, medium and high GC content, respectively; Supplementary Fig. S15 ). MRE-chip showed a substantially weaker overall correlation with mTAG-seq ( r =0.44). Consistent with the ability of mTAG to enrich for unmethylated genomic regions, the relative mTAG-seq density in the brain throughout different gene-associated regions showed inverse features compared with modified cytosine maps generated by bisulfite-sequencing of the H1 cell line [3] ( Fig. 5a ). At the level of individual genes, mTAG-seq profiles of typical protein coding genes showed that the promoters and CpG islands were unmethylated, consistent with high MRE-seq and no MeDIP-seq signal ( Fig. 5b ). We also demonstrated that the mTAG approach can identify and map the unmodified genomic retroelements. L2b, a non-long terminal repeat retrotransposon (chr19: 41257434–41257808, 11 CpGs), appeared to be unmethylated in the brain as supported by the lack of MeDIP reads and a detectable peak in the MRE profile ( Fig. 5c ). Another example, MLT1B—a mammalian long terminal repeat retrotransposon (chr14: 106804419–106804800, 3 CpGs), was not detectable by MRE due to the scarcity of suitable restriction endonuclease sites and had a very weak MeDIP signal ( Fig. 5c ). In both cases, strong mTAG signals illustrated a positive display of these fairly abundant differentially modified DNA retroelements. A more complex situation is shown in Fig. 5d where seven SINE elements were marked by both mTAG-seq and MeDIP-seq in the brain samples, suggesting their intra-individual epigenetic variation. 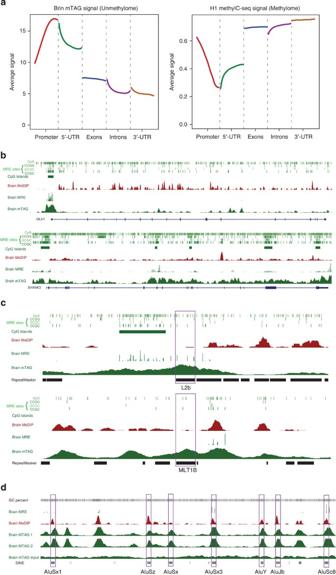Figure 5: Epigenomic mTAG-seq profiles of human brain DNA. (a) mTAG-seq and MethylC-seq profiles over a mega-gene. Left, mTAG-seq signal density (unmethylome) displayed with GenePlot50throughout different gene-associated regions. Gene annotations were obtained from UCSC Genome Browser. Promoter was defined as 1 kb upstream from transcript start site. Promoters, transcription start sites and 5′-UTRs all displayed increased mTAG-seq signal compared with gene bodies, consistent with hypomethylation of these regions. Right, MethylC-seq profile (methylome) of H1 human embryonic stem cells over a composite gene (replot ofFig. 3afrom Listeret al.3). (b) mTAG-seq profile of two typical protein coding genes. Genome browser view of mTAG-seq data over typical genes in comparison to MeDIP-seq and MRE-seq of the brain51. The upper panel displayedMLH1, and the lower panel displayedSHANK3. Promoters of both genes were unmethylated, consistent with high mTAG-seq, high MRE-seq, and no MeDIP-seq signal. The gene body ofSHANK3contained several unmethylated CpG islands, which exhibited high mTAG-seq signal. (c) Unmethylated retroelements revealed by mTAG-seq. Genome browser view of two retroelements. The upper panel displayedL2b. The element was marked by high mTAG-seq, high MRE-seq and low MeDIP-seq signal. These three methods were in agreement in supporting the unmethylated status of the element. The lower panel displayedMLT1B. The element was marked by high mTAG-seq and low MeDIP-seq signal, indicating a hypomethylated status. MRE-seq produced no signal over this region due to the low abundance of restriction endonuclease sites. (d) Partially methylated retroelements revealed by mTAG-seq. Genome browser view of seven SINE elements. These elements were consistently marked by mTAG-seq in two brain samples;the same elements displayed a MeDIP-seq signal, altogether suggesting they were partially methylated (contained both unmodified and methylated CpGs). A non-enriched input track (mTAG Input) was also shown indicating that the coenrichment of the MeDIP-seq and mTAG-seq signals over these SINE element was not an artifact of sequence alignment. Figure 5: Epigenomic mTAG-seq profiles of human brain DNA. ( a ) mTAG-seq and MethylC-seq profiles over a mega-gene. Left, mTAG-seq signal density (unmethylome) displayed with GenePlot [50] throughout different gene-associated regions. Gene annotations were obtained from UCSC Genome Browser. Promoter was defined as 1 kb upstream from transcript start site. Promoters, transcription start sites and 5′-UTRs all displayed increased mTAG-seq signal compared with gene bodies, consistent with hypomethylation of these regions. Right, MethylC-seq profile (methylome) of H1 human embryonic stem cells over a composite gene (replot of Fig. 3a from Lister et al. [3] ). ( b ) mTAG-seq profile of two typical protein coding genes. Genome browser view of mTAG-seq data over typical genes in comparison to MeDIP-seq and MRE-seq of the brain [51] . The upper panel displayed MLH1 , and the lower panel displayed SHANK3 . Promoters of both genes were unmethylated, consistent with high mTAG-seq, high MRE-seq, and no MeDIP-seq signal. The gene body of SHANK3 contained several unmethylated CpG islands, which exhibited high mTAG-seq signal. ( c ) Unmethylated retroelements revealed by mTAG-seq. Genome browser view of two retroelements. The upper panel displayed L2b . The element was marked by high mTAG-seq, high MRE-seq and low MeDIP-seq signal. These three methods were in agreement in supporting the unmethylated status of the element. The lower panel displayed MLT1B . The element was marked by high mTAG-seq and low MeDIP-seq signal, indicating a hypomethylated status. MRE-seq produced no signal over this region due to the low abundance of restriction endonuclease sites. ( d ) Partially methylated retroelements revealed by mTAG-seq. Genome browser view of seven SINE elements. These elements were consistently marked by mTAG-seq in two brain samples;the same elements displayed a MeDIP-seq signal, altogether suggesting they were partially methylated (contained both unmodified and methylated CpGs). A non-enriched input track (mTAG Input) was also shown indicating that the coenrichment of the MeDIP-seq and mTAG-seq signals over these SINE element was not an artifact of sequence alignment. Full size image Here we describe the first approach for covalent capture and mapping of the DNA unmethylome. As unmodified cytosines represent a smaller proportion of CpG sites compared with methylated ones (depending on the tissue, over 70% of cytosines in the human genome are methylated [29] ), analysis of this smaller, unmethylated DNA fraction may reduce the number of statistical comparisons and is more sensitive for detecting subtle epigenetic changes [5] . Taking also into account, the occurence of the other modified cytosines (hmC, fC, caC), which cannot be easily differentiated from mC and C, our approach provides a unique cross-section through the complex chemical landscape of the mammalian epigenome. Furthermore, MeDIP and MBD enrichment have been noted to have a substantial CpG coverage bias towards the highly methylated sequences [16] , [17] , [31] . Based on our decile correlation analyses, mTAG shows its strength in low and intermediate CpG density genomic regions, which comprise >80% of the genome and over 50% of all CpG sites, and which are insufficiently covered by the existing techniques. Such regions include enhancer elements, CpG island shores and promoters of cell type-specific genes, which often undergo dramatic changes in CpG modification status during cell differentiation and development [39] , [40] , [41] , [42] , and which are candidate markers of diseases such as cancer [43] . Moreover, mTAG can be considered not only as a powerful and cost-effective alternative, but also as a complementary technique to 5mC-specific methods such as MeDIP and, likely, to a newly described covalent method, TAmC-seq [33] . mTAG-seq profiling permitted positive identification of unmethylated and partially methylated transposable elements, which are often left behind using MRE and MeDIP analyses. Although transposons and repetitive elements are commonly thought to be heavily methylated [3] , [44] , some of them show a loss in methylation in cancer [45] or in response to other developmental cues, and may thus be of high predictive and diagnostic value. The input quantity of human gDNA (100–300 ng) required for whole-genome mTAG analysis was at the lower end of typical samples consumed for MethylC-seq (5 μg), MeDIP-seq (0.1–5, typically >1 μg) or MethylCap-seq or MBD-seq (1–3 μg) [46] , [47] , owing to the covalent labelling, tight affinity capture and mild chemical release employed in the enrichment procedure. The analytical procedure is robust and well adaptable for high-throughput epigenomic studies. Both the conventional and click versions of the method allow for efficient unmethylome analyses, although due to its very low nonspecific labelling, the latter appears to be the method of choice for large-scale populational studies. The mTAG technology thus brings a new analytical platform with its follow-up application-driven modalities, providing a valuable addition to the toolbox of epigenomic studies. AdoMet analogues AdoMet analogues ( Supplementary Fig. S1a ) were obtained by S-selective coupling of 4-nitrophenylsulfonyl-activated side chains to S -adenosyl- L -homocysteine [26] . Ado-6-amine was isolated as a diastereomeric mixture containing ~50% of the enzymatically active S,S -diasteromer. For Ado-6-azide, the enzymatically active diasteromer was isolated by reversed-phase HPLC. Genomic DNA DNA from sperm and post-mortem (prefrontal cortex) human brains were purified using standard phenol–chloroform extraction. Human fibroblast IMR90 gDNA was kindly provided by R. Lister or obtained from the UK Health Protection Agency. Brain samples were received from the Harvard Brain Tissue Resource Center. Sperm samples were collected at the Krembil Family Epigenetics laboratory, Centre for Addiction and Mental Health, Toronto. Centre for Addiction and Mental Health Research Ethics Office approved the study under the protocol number 175-2009. All of the patients and relatives gave informed consent for the use of tissues. qPCR analysis DNA probes for qPCR monitoring of DNA recovery were prepared by PCR amplification of C57BL/6 mouse gDNA with corresponding primers (Sp-PCR-dir, 5′-GTGTTGGGGTGACTATTATGAND-3′ Sp-PCR-rev, 5′-CCTATACTCAGCGCATCC-3′ for the specific probe, and Ns-PCR-dir, 5′-GCCCACTTCACTTCTTGTGAND-3′ Ns-PCR-rev, 5′-AGGCCAAAAGAAAGAAGAGAT-3′ for the nonspecific one). Reverse transcriptase PCR experiments were performed with a Rotor-Gene 6000 real-time PCR system (Corbett Research) using a Maxima Probe qPCR Master Mix (ThermoFisher). Primers (0.3 μM)for the specific DNA fragment, 1 μM primers for the nonspecific probe and 250 nM of the respective dual-labelled probe were used in each reaction. The amplification program was set as: 95 °C for 10 min, 40 cycles 95 °C for 15 s, 60 °C for 1 min. Primer sequences are listed in Supplementary Table S2 . mTAG-directed biotin labelling and enrichment of DNA gDNA was sonicated on a Bioruptor UCD-200 (Diagenode) in EB buffer (10 mM Tris-HCl (pH 8.5) for 2 h to yield fragments with a peak size of 250 bp. Sheared DNA was end-filled using the DNA End Repair Kit (ThermoFisher) and DNA was purified using a QIAquick Nucleotide Removal kit (Qiagen). For mTAG labelling using amine-NHS chemistry, reactions of 25 μl contained 100–300 ng of sheared and blunt-ended gDNA (and optionally 50 ng of qPCR reference fragments), 50 μM of freshly diluted cofactor analogue Ado-6-amine and engineered eM.SssI (no enzyme for 0% labelling intensity; 45 nM for Low labelling intensity; 180 nM for Medium labelling, or 1440, nM for High labelling) in M.SssI reaction buffer (10 mM Tris-HCl pH 7.6, 50 mM NaCl, 0.1 mg ml −1 ). Reactions were incubated at 37 °C for 30 or 60 min, followed by heating at 65 °C for 15 min. DNA samples were purified using a QIAquick Nucleotide Removal kit and treated with 8.6 mM biotin disulphide N-hydroxysuccinimide ester (NHS-SS-biotin, Sigma) in 0.15 M sodium bicarbonate (pH 9.0) at room temperature for 2.5 h, and again purified with a QIAquick Nucleotide Removal kit. For mTAG-click labelling using azide-alkyne conjugation, 25 μM Ado-6-azide cofactor and eM.SssI (90 nM for Medium labelling, or 180 nM for High labelling) were used. Reactions were incubated at 37 °C for 30 or 60 min, followed by heating at 80 °C for 10 min. Dibenzylcyclooctyne-SS-PEG11-Biotin or dibenzylcyclooctyne-SS-PEG3-BiotinConjugate (Jena Bioscience) was then added to 0.2 mM concentration and incubated at 37 °C for 2 h. The mixture of the Dynabeads MyOneC1 Streptavidin (0.1 mg) and DNA recovered after biotinylation step were incubated in 10 mM Tris-HCl (pH 8.5), 1 M NaCl buffer at room temperature for 3 h on a roller. Beads were washed 3 × with washing buffer A (10 mM Tris-HCl (pH 8.5), 3 M NaCl); 2 × with washing buffer B (10 mM Tris-HCl (pH 8.5), 1 M NaCl) and finally resuspended in 100 mM Tris-HCl pH 7.4. For recovery of enriched DNA fraction, DNA-bound beads were incubated in 200 mM DTT at room temperature for 1 h, and released DNA was precipitated with propanol-2. DNA pellet was resuspended in 9 μl of 1xT4 DNA Ligase buffer (ThermoFisher) and ligated to double-stranded adaptors as indicated below. PCR amplification of enriched DNA for microarray analysis PCR adaptors were prepared by annealing equal amounts (100 μM) of single-stranded oligonucleotides A-25 (5′-AGTTACATCTTGTAGTCAGTCTCCA)-3′ and A-19 (5′-TGGAGACTGACTACAAGAT)-3′ in T4 DNA Ligase buffer. To ligate adaptors to gDNA fragments, DNA recovered from beads was incubated with 5 μM adaptors at 45 °C for 10 min, the mixture was chilled on ice and after addition of 5 a.u. of T4 DNA Ligase (ThermoFisher) was further incubated at 22 °C overnight. For PCR amplification, adaptor-ligated DNA was incubated with 100 mM 2-mercaptoethanol for 10 min at room temperature (to preclude inadvertent formation of inter-nucleotide disulphide cross-links), followed by PCR in Taq Buffer with (NH 4 ) 2 SO 4 supplemented with 0.2 mM deoxyribonucleotide (dNTP), 1 mM MgCl 2 , 1 μM A-25 oligonucleotide and 5 a.u. Taq DNA Polymerase (ThermoFisher). PCR cycling conditions: 1 min 50 °C, 5 min 72 °C, 4 min 94 °C, 15 cycles of 1 min 94 °C, 1 min 65 °C, 1 min 72 °C and the final extension step is at 72 °C for 2 min. For mTAG-click-labelled DNA, the extension step of the first cycle was prolonged to 5 min to alleviate the possible impairment of PCR amplification because of bulky groups left on DNA (see Fig. 1 ). Microarray analysis For microarry hybridization experiments,an aliquot of 1/10 the above amplified DNA sample was used as template in a second-round PCR that contained dUTP as specified in the WT Double-Stranded DNA Terminal Labelling Kit (Affymetrix). The reaction was carried out with 200 pmol of adaptor-specific A-25 primer, 2.5 mM MgCl 2 , 0.4 mM dNTPs with 0.02 mM dUTP, and 5 a.u. Taq polymerase (New England Biolabs). The PCR amplifications were performed at 95 °C for 1 min followed by 15 cycles of 94 °C for 15 s, 65 °C for 30 s and 1 min at 72 °C, with an extension of 5 s at the last step of each subsequent cycle. For the microarray hybridization, 9 μg of purified uracil-containing amplicons were fragmented to 50–100 bp using GeneChip Double-stranded DNA Terminal Labelling kit (Affymetrix). Individual samples were hybridized to a separate GeneChip Human Tiling 2.0 R Arrays. The arrays were washed, stained and scanned using an Affymetrix GeneChip Scanner as described in the Affymetrix ChIP Assay protocol. Array data was quantile normalized, and mTAG log ratios for unlabelled (0% labelling) over labelled (5–80% labelling) probes were generated. MeDIP analysis [6] of IMR90 gDNA was performed as follows. Two replicate samples were prepared using the MagMeDIP kit (Diagenode) according the manufacturer’s instructions. An aliquote of each sample was used as a template in two independent PCR reactions to confirm enrichment of methylated and depletion of unmethylated sequences, relative to fragmented input DNA. The enriched samples were further amplified using a WGA kit (Sigma) and analysed on microarrays as described. Comparisons between MeDIP-chip and mTAG-chip gDNA from three brain and five sperm samples were processed in a mTAG and MeDIP protocol (three replicates per sample and protocol). Steps 1–5 of mTAG enrichment were performed as described in the high-throughput mTAG-click protocol ( Supplementary Methods ). Samples in 50 mM DTT, 60 mM Tris pH 7.8 were dA-tailed in a reaction containing 0.2 mM dATP, 5 mM MgCl 2 , 5 mM Tris pH 7.8 and 5 a.u. Klenow, exo- (Thermo Scientific). Aten-fold molar excess of adaptor was ligated to DNA fragments. Adaptors had been prepared by annealing equimolar amounts of each primer (Ad1, 5′-[phos]-GATCGGAAGAGCACACGTCT-3′ and Ad2, 5′-ACACTCTTTCCCTACACGACGCTCTTCCGATCT)-3′. Ligation of adaptors to the DNA fragment was performed overnight at 22 °C in a 30 μl volume in Buffer (6 mM MgCl 2 , 0.5 mM ATP) and 10 a.u. T4 DNA ligase. Purification of samples was completed with the ZR-96 DNA Clean & Concentrator-5 kit (Zymo Research). Samples were then incubated with 32 mM 2-mercaptoethanol for 10 min at room temperature. PCR amplification was performed in two rounds. Initially, samples were combined with buffer (75 mM Tris-HCl (pH 8.8), 20 mM (NH 4 ) 2 SO 4 , 0.01% Tween 20), 1 mM MgCl 2 , 200 μM dNTPs, 0.5 μM of each primer (Ad-F, 5′-AATGATACGGCGACCACCGAGATCTACACTCTTTCCCTACACGACGCTCTTCCGATCT-3′, Ad-R, 5′-GTGACTGGAGTTCAGACGTGTGCTCTTCCGATCT)-3′ and 6.3 a.u. Taq polymerase (ThermoFisher) in a reaction volume of 100 μl. The second PCR step (using the Ad-F and Ad-R primers) and PCR cycling conditions were performed as described in the high-throughput mTAG-click protocol. In the MeDIP experiment, samples were dA-tailed and ligated to the same adaptors. Ligated DNA was purified with Ampure XP beads (Agencourt). Approximately 800 ng of each sample, including antibody negative controls, were processed using the MagMeDIP kit (Diagenode), following the manufacturer’s instructions. Kit internal controls were evaluated using qPCR, and all MeDIP samples indicated a specificity that exceeded 98%. MeDIP-treated samples were then PCR-amplified in a two-step procedure (10 PCR cycles in step one and 6 PCR cycles in step two) as in the mTAG approach described above. MeDIP and mTAG samples were normalized separately as follows. First, interarray correlations (IACs) were assessed to identify and remove outlying samples [48] . Log2 scaled raw intensity values of samples were correlated with one another. These IACs were averaged for each array and compared with the resulting distribution of IACs. Samples with an average IAC of more than two s.d. values below the mean IAC were considered outliers and removed in repeat cycles. Next, samples were quantile normalized, mean total input was subtracted and probes from repetitive regions were removed. Adjacent probes were smoothed using 3.1 kb Gaussian kernel. To assess the clustering of samples, 300,000 most variable probes among mTAG and MeDIP samples were selected separately and their union was used. Distance between samples was defined as inverse of a scaled Pearson correlation. Hierarchical clustering with average linkage was employed to produce the clustering dendrogram. Average Pearson correlation of matching MeDIP and mTAG samples was quantified using 20% most intense probes. mTAG-seq Nine brain samples (from eight different individuals plus one technical replicate) were sheared at an average length of 300 bp and labelled using the mTAG approach as described in the high-throughput mTAG-click protocol. The purified mTAG-enriched samples, along with a sheared aliquot of a sample that was not enriched in the mTAG procedure (total input), were then submitted to the Beijing Genomics Institute (BGI) for final library preparation and sequencing. Library preparation involving adenylation of 3′-ends, adaptor ligation and PCR amplification with unique index primers was performed as described in the Illumina Multiplexing Sample Preparation Oligonucleotide kit. The only changes to this library preparation protocol were that the samples were treated with 10 mM 2-mercaptoethanol for 10 min at room temperature before PCR amplification, and only 14 cycles of PCR were performed. Paired-end sequencing was completed on an Illumina HiSeq platform generating ~100 million paired-end reads for each mTAG-seq library, with a read length of 90 bp. These reads were mapped to the human genome assembly hg19 using BWA [49] with default parameters. Sequencing reads from female samples were mapped to the same reference with chromosome Y excluded. Alignments with mapping quality score greater or equal to 10 were considered unique alignments. Alignments mapped to exactly the same genomic location were considered as redundant reads resulted from PCR amplification and were removed from further analysis. The non-redundant, uniquely mapped sequence fragments were further processed using in house tool iteres ( http://epigenome.wustl.edu/iteres/ ) to generate read density files. These read density files were uploaded to both the UCSC Genome Browser ( http://genome.ucsc.edu ) and the Washington University Epigenome Browser ( http://epigenomegateway.wustl.edu ) for visualization and further analysis. Accession codes : Microarray data have been deposited in the NCBI Gene Expression Omnibus under accession codes GSE36305 . How to cite this article: Kriukienė, E. et al. DNA unmethylome profiling by covalent capture of CpG sites. Nat. Commun. 4:2190 doi: 10.1038/ncomms3190 (2013)